Loss of TRPM2 function protects against irradiation-induced salivary gland dysfunction Xerostomia as a result of salivary gland damage is a permanent and debilitating side effect of radiotherapy for head and neck cancers. Effective treatments for protecting, or restoring, salivary gland function are not available. Here we report that irradiation treatment leads to activation of the calcium-permeable channel, transient potential melastatin-like 2 (TRPM2), via stimulation of poly-ADP-ribose polymerase. Importantly, irradiation induced an irreversible loss of salivary gland fluid secretion in TRPM2+/+ mice while a transient loss was seen in TRPM2−/− mice with >60% recovery by 30 days after irradiation. Treatment of TRPM2+/+ mice with the free radical scavenger Tempol or the PARP1 inhibitor 3-aminobenzamide attenuated irradiation-induced activation of TRPM2 and induced significant recovery of salivary fluid secretion. Furthermore, TPL (4-hydroxy-2,2,6,6-tetramethylpiperidine- N -oxyl) induced complete recovery of function in irradiated TRPM2−/− mice. These novel data demonstrate that TRPM2 is activated by irradiation, via PARP1 activation, and contributes to irreversible loss of salivary gland function. More than 40,000 new cases of head and neck cancer are reported in the United States per year and >350,000 worldwide [1] . Radiotherapy is still the primary mode of treatment for majority of the patients, delivered alone or in combination with surgery and/or chemotherapy [2] , [3] , [4] , [5] . However, irradiation (IR) causes significant acute- and long-term, either direct or by-stander, effects on other healthy tissues that are in the field of treatment. A debilitating side effect of IR in head and neck cancer patients is xerostomia, or dry mouth, a consequence of decreased saliva secretion due to persistent, irreversible, loss of salivary gland function. Early effects of IR could be induced by membrane damage while more delayed and long-term effects have been proposed to be a consequence of IR-induced damage of progenitor cells within the adult salivary gland, which leads to a compromise in the regenerative capacity of the gland [6] , [7] , [8] , [9] , [10] . Owing to the slow turnover rate of cells (60–120 days) within the gland, loss of tissue occurs slowly. However, in many cases, significant changes are seen in the quantity and composition of saliva before overt damage or loss of gland is detected. This is more obvious in mice where the onset of fibrosis and loss of salivary gland tissue (more specifically acinar cells) is relatively slow [11] . The mechanism underlying the IR-induced salivary hypofunction in glands that have apparently normal morphology is not yet understood. Nevertheless, it is clear that loss of salivary gland fluid secretion is the causative factor in xerostomia, which leads to a marked decline in quality of life for the patients post therapy, even when the tumour itself has been controlled [4] , [5] , [12] . No adequate therapies are currently available to protect against, or reverse, IR-induced salivary hypofunction. Most treatment options are essentially palliative in nature [13] , [14] , [15] . Transient Potential Melastatin-like 2 (TRPM2) is a Ca 2+ -permeable non-selective cation channel that has been suggested to be a redox-sensor [16] . The channel is activated by H 2 O 2 and other agents/conditions that produce reactive oxygen species (ROS) [17] . Recently, TRPM2 channels have attracted interest as a potential target for pathogenic processes that are characterized by an increased oxidative microenvironment [18] . TRPM2 has a unique C-terminal adenosine diphosphate ribose (ADPR) pyrophosphatase domain (Nudix-like domain or NUDT9 homology domain). Binding of ADPR to NUDT9-H activates the channel and so conditions that lead to poly-ADP-ribose polymerase (PARP) activation result in generation of ADPR and gating of the channel [17] . IR leads to generation of ROS, which has been implicated in the mechanism of salivary gland damage and impairment of fluid secretion. Further, DNA damage as a result of IR can lead to PARP activation and ADPR generation [19] . Here we report that TRPM2 is present salivary gland cells and is activated by IR. While irradiated (15 Gy, 1 dose) TRPM2+/+ mice display an irreversible loss of salivary gland fluid secretion within 10 days after IR, mice lacking TRPM2 show a transient loss, which recovers to >60% of the normal saliva flow within a month after treatment. Treatment of mice before IR with TPL (4-hydroxy-2,2,6,6-tetramethylpiperidine- N -oxyl), a free radical scavenger, or 3-AB, a PARP1 inhibitor, reduce activation of TRPM2 and exert significant protection of salivary gland function, suggesting that IR-activation of TRPM2 is mediated via generation of ROS and PARP1 activation. Together, our findings provide evidence that TRPM2 contributes to IR-induced salivary gland dysfunction. Functional TRPM2 channels are present in HSG cells Treatment of HSG cells with H 2 O 2 resulted in a rapid and sustained increase of intracellular [Ca 2+ ] ([Ca 2+ ] i ) ( Fig. 1a ), which was reduced and transient when cells were treated in medium without Ca 2+ , suggesting that the sustained [Ca 2+ ] i increase was largely due to Ca 2+ influx with a small intracellular Ca 2+ release component. Further, H 2 O 2 triggered the activation of membrane conductance ( Fig. 1b ) with maximum current amplitude (26.5±5.7 pA/pF) reached within 30–60 s. The I-V relationship of the current was relatively linear and similar to that reported for TRPM2 [17] . A cation current was also activated by inclusion of ADPR, the specific agonist of TRPM2, in the pipette solution (current density=23.9±6.3 pA/pF, Fig. 1d ) with I-V relationship similar to that generated by H 2 O 2 ( Fig. 1e ). The ADPR-activated membrane current was sensitive to clotrimazole a widely used, although not very specific, TRPM2 channel inhibitor ( Fig. 1f ). siTRPM2 was used to decrease channel expression in HSG cells ( Fig. 1g and Supplementary Fig. S1 , siTRPM2#1 was used in the studies described below). Knockdown of TRPM2 induced a significant decrease ( Fig. 1h ) in H 2 O 2 -induced Ca 2+ influx (0.45±0.09 and 0.17±0.02 in control and siTRPM2 cells, respectively), without any effect on intracellular Ca 2+ release. More specifically, siTRPM2 decreased ADPR-stimulated membrane conductance ( Fig. 1i ). Average current density decreased from 22±3.1 in control cells to 14±4 pA/pF in siTRPM2-treated cells ( P <0.01). In aggregate, the findings presented in Fig. 1 provide evidence for the presence of functional TRPM2 channels in the human submandibular gland cell line, HSG. 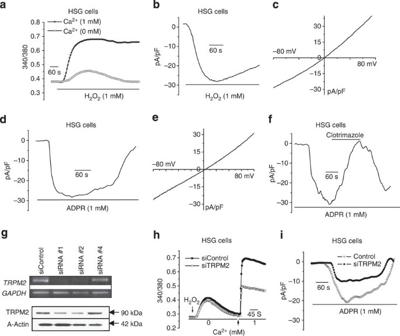Figure 1: Activation of TRPM2 in HSG cells. TRPM2 activity was assessed either by measuring fura2 fluorescence changes (340/380 ratio) or by whole-cell patch-clamp measurements in HSG cells. (a) Fura 2 fluorescence measurements in HSG cells treated with H2O2in the presence and absence of Ca2+in the external medium. (b) Development of cation currents following H2O2treatment. (c) I-V relationship of maximum current inb. (d–e) Similar patch-clamp measurements with ADPR included in the pipette solution. (f) Sensitivity of ADPR-induced current to 50 μM clotrimazole. Effect of siTRPM2 on TRPM2 transcript (upper panel) and protein (lower panel). (h,i) Effect of siTRPM2 on H2O2-induced intracellular Ca2+release and Ca2+influx and ADPR-induced cation currents, respectively. All other experimental details are provided in the methods section. These are representative traces from multiple experiments. Figure 1: Activation of TRPM2 in HSG cells. TRPM2 activity was assessed either by measuring fura2 fluorescence changes (340/380 ratio) or by whole-cell patch-clamp measurements in HSG cells. ( a ) Fura 2 fluorescence measurements in HSG cells treated with H 2 O 2 in the presence and absence of Ca 2+ in the external medium. ( b ) Development of cation currents following H 2 O 2 treatment. ( c ) I-V relationship of maximum current in b . ( d – e ) Similar patch-clamp measurements with ADPR included in the pipette solution. ( f ) Sensitivity of ADPR-induced current to 50 μM clotrimazole. Effect of siTRPM2 on TRPM2 transcript (upper panel) and protein (lower panel). ( h , i ) Effect of siTRPM2 on H 2 O 2 -induced intracellular Ca 2+ release and Ca 2+ influx and ADPR-induced cation currents, respectively. All other experimental details are provided in the methods section. These are representative traces from multiple experiments. Full size image TRPM2 is activated by IR in HSG cells HSG cells were subjected to IR (15Gy) and [Ca 2+ ] i was monitored 45 min later. Addition of external Ca 2+ to IR cells in a Ca 2+ -free medium induced a rapid rise in [Ca 2+ ] i that was significantly greater than that in control, non-IR cells ( Fig. 2a ). There was no significant difference between the [Ca 2+ ] i in cells in the absence of external Ca 2+ . Knockdown of TRPM2 reduced Ca 2+ influx triggered by IR to levels similar to that in non-IR cells ( Fig. 2b ). Further, knockdown of TRPM2 also decreased initial HSG cell damage following IR. About 80% of HSG cells treated with control siRNA displayed uptake of trypan blue compared with about 40% in siTRPM2-treated HSG cells and <2% in non-IR cells ( Fig. 2d–f ). The percentage of viable cells in siTRPM2 group 96 h after IR was about three times more (58.7±7.1%) than in the control group (18.3±1.6%, P <0.001). Therefore, our data suggest that TRPM2 is activated by IR of a human submandibular gland cell line and has an essential role in IR-induced cellular damage. 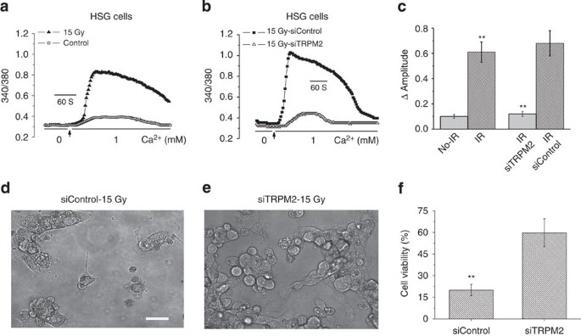Figure 2: Activation of TRPM2 by IR of HSG cells and effect on cell viability. (a) [Ca2+]Imeasurements in HSG cells (control and subjected to 15 Gy radiation treatment). Measurements were made within 45–90 min after IR. Point of inclusion of Ca2+to the external medium is indicated in the Fig. (b) Effect of siTRPM2 on radiation-induced increase in [Ca2+]i. (c) Average increase in [Ca2+]I(above baseline in the experiments shown in andaandb). Values marked **represent a significant difference (P<0.01, no. of cells tested are from 275–320) from the respective controls in each experiment. (d–f) Effect of IR on cell viability assessed based on Trypan Blue exclusion in HSG cells 96 h after 15 Gy radiation. Cells were stained with Trypan Blue and counted. Images of control-IR and siTRPM2-IR are shown indande. Scale bar, 20 μm. Average number of viable cells in the two groups are given inf. **Indicates a significant difference (P<0.01) in the value compared with the control condition. Figure 2: Activation of TRPM2 by IR of HSG cells and effect on cell viability. ( a ) [Ca 2+ ] I measurements in HSG cells (control and subjected to 15 Gy radiation treatment). Measurements were made within 45–90 min after IR. Point of inclusion of Ca 2+ to the external medium is indicated in the Fig. ( b ) Effect of siTRPM2 on radiation-induced increase in [Ca 2+ ] i . ( c ) Average increase in [Ca 2+ ] I (above baseline in the experiments shown in and a and b ). Values marked **represent a significant difference ( P <0.01, no. of cells tested are from 275–320) from the respective controls in each experiment. ( d – f ) Effect of IR on cell viability assessed based on Trypan Blue exclusion in HSG cells 96 h after 15 Gy radiation. Cells were stained with Trypan Blue and counted. Images of control-IR and siTRPM2-IR are shown in d and e . Scale bar, 20 μm. Average number of viable cells in the two groups are given in f . **Indicates a significant difference ( P <0.01) in the value compared with the control condition. Full size image IR activates TRPM2 in acinar cells The physiological relevance of TRPM2 in salivary gland acinar cells was demonstrated by assessing channel function in freshly dispersed single mouse submandibular gland acinar cells. H 2 O 2 and ADPR-activated non-selective cation currents that were similar to those measured in HSG cells ( Fig. 3a–d ). H 2 O 2 also increased [Ca 2+ ] i in acinar cells, the magnitude of which was higher and more sustained the presence of external Ca 2+ than in a Ca 2+ -free medium where a small transient response was seen ( Fig. 3e ). To confirm activation of TRPM2 by IR, mice were subjected to 15 Gy-IR targeted to salivary glands ( Supplementary Fig. S2 ) and 24 h later submandibular glands were excised and acini were prepared. A relatively high constitutive Ca 2+ influx was seen in cells from irradiated mice, compared with those from glands in control mice ( Fig. 3f ). 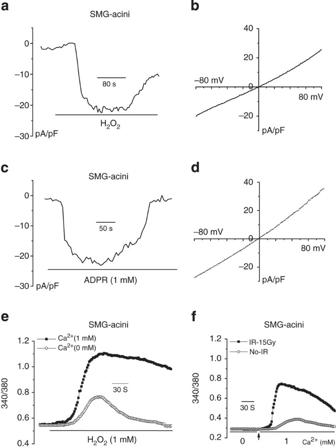Figure 3: TRPM2 channels exist in mouse submandibular gland acini (SMG) and are activated by IR. Dispersed single acinar cells from mouse submandibular glands were prepared as described in the methods section and used for [Ca2+]ior whole-cell patch-clamp measurements. (a,c) Cation channel activity induced by H2O2and ADPR (included in the pipette solution), respectively. I-V relationships of the currents inaandcare shown in (b,d). (e) H2O2-induced [Ca2+]iincrease in fura-2-loaded acinar cell in the presence or absence of external Ca2+. (f) Constitutive Ca2+influx activity in acini from mouse submandibular glands that were excised 24 h after IR of the animals (see details in Methods section). Presence of Ca2+in the external medium is indicated in the Fig. Figure 3: TRPM2 channels exist in mouse submandibular gland acini (SMG) and are activated by IR. Dispersed single acinar cells from mouse submandibular glands were prepared as described in the methods section and used for [Ca 2+ ] i or whole-cell patch-clamp measurements. ( a , c ) Cation channel activity induced by H 2 O 2 and ADPR (included in the pipette solution), respectively. I-V relationships of the currents in a and c are shown in ( b , d ). ( e ) H 2 O 2 -induced [Ca 2+ ] i increase in fura-2-loaded acinar cell in the presence or absence of external Ca 2+ . ( f ) Constitutive Ca 2+ influx activity in acini from mouse submandibular glands that were excised 24 h after IR of the animals (see details in Methods section). Presence of Ca 2+ in the external medium is indicated in the Fig. Full size image Salivary fluid secretion recovers in TRPM2−/− mice after IR H 2 O 2 -induced [Ca 2+ ] i elevation was significantly lower in submandibular gland acini from TRPM2−/− mice compared with that in cells from TRPM2+/+ mice ( Fig. 4a ). To examine the effects of IR on TRPM2, both sets of mice were treated with radiation (15 Gy) and 24 h later, submandibular glands were excised, acinar cells were isolated and used for [Ca 2+ ] i measurements. Constitutive activation of Ca 2+ entry was seen in acinar cells from TRPM2+/+ mice after IR. Ca 2+ entry was significantly lower (>80%) in cells isolated from IR-TRPM2−/− mice ( Fig. 4b ). These data firmly establish that IR induces activation of Ca 2+ influx via TRPM2. Supplementary Fig. S1 shows the genotyping (A) of the mice and the loss of TRPM2 expression in submandibular glands from TRPM2−/− by western blotting (B), as well as by immunofluorescence (D). TRPM2 was detected in acinar and ductal cells in samples from TRPM2+/+ mice. 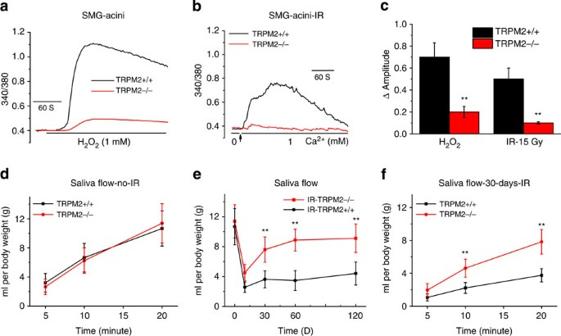Figure 4: Radiation-induced loss of salivary fluid secretion is absent in TRPM2−/− mice. (a) H2O2-induced increases in [Ca2+]iin SMG acini from TRPM2+/+ and TRPM2−/− mice. (b) IR-induced increase in constitutive Ca2+influx in TRPM2+/+ and TRPM2−/− mice. (c) Average data from the experiments shown inaandb. **Indicates values with statistically significant difference compared with the unmarked values in each experiment (number of cells tested from 175–205 per group). Mice were treated with the muscarinic agonist, pilocarpine (0.5 mg kg−1, subcutaneous injection) and saliva flow was collected (details given in the Methods section) in TRPM2+/+ and TRPM2−/− mice before IR (dshows saliva secretion over a 20-min collection period), on different days after 15 Gy IR (eup to 120 days); and over a 20-min time point 30 days after IR (f). **Indicates significant difference,P<0.01, between the corresponding values in TRPM2+/+ mice (10–11 animals per group). All values in (c–f) are defined as mean±s.e. Figure 4: Radiation-induced loss of salivary fluid secretion is absent in TRPM2−/− mice. ( a ) H 2 O 2 -induced increases in [Ca 2+ ] i in SMG acini from TRPM2+/+ and TRPM2−/− mice. ( b ) IR-induced increase in constitutive Ca 2+ influx in TRPM2+/+ and TRPM2−/− mice. ( c ) Average data from the experiments shown in a and b . **Indicates values with statistically significant difference compared with the unmarked values in each experiment (number of cells tested from 175–205 per group). Mice were treated with the muscarinic agonist, pilocarpine (0.5 mg kg −1 , subcutaneous injection) and saliva flow was collected (details given in the Methods section) in TRPM2+/+ and TRPM2−/− mice before IR ( d shows saliva secretion over a 20-min collection period), on different days after 15 Gy IR ( e up to 120 days); and over a 20-min time point 30 days after IR ( f ). **Indicates significant difference, P <0.01, between the corresponding values in TRPM2+/+ mice (10–11 animals per group). All values in ( c – f ) are defined as mean±s.e. Full size image Salivary gland fluid secretion in TRPM2+/+ and −/− mice, measured following subcutaneous injection with pilocarpine (0.5 mg kg −1 ), demonstrated no significant differences in the two sets of animals before radiation ( Fig. 4d ). However, 10 days after IR, the saliva flow in both sets of mice was significantly reduced compared with the respective values before IR. Notably, fluid secretion in TRPM2−/− mice was about 20% greater than that in TRPM2+/+ mice, which retained only about 30% of the secretion seen before IR. Importantly, saliva secretion in IR-TRPM2−/− mice displayed significant recovery to about 60% of initial level by 30 days after IR and to 70% of the initial level by 60 days. In contrast, salivary flow in TRPM2−/− mice remained at about 30% of the initial level for the length of the experiment up to 4 months ( Fig. 4e ). Saliva flow rate in TRPM2−/− mice was higher compared with that in TRPM2+/+ mice 30 days after IR ( Fig. 4f ). Saliva secretion did not change during this time period in mice that did not receive IR. Together the data in Fig. 4 demonstrate that IR induces a transient loss of salivary fluid secretion in TRPM2−/− mice, whereas it triggers an irreversible loss of function in TRPM2+/+ mice. As IR-induced activation of TRPM2 was eliminated in TRPM2−/− mice, we suggest that the transient loss of function seen in TRPM2−/− mice is indicative of effects that are independent of channel function, likely induced by direct effects of IR or IR-generated ROS. Note that under our conditions of radiation and post-IR maintenance (see Methods for details) no significant health issues were observed in the animals up to 4 months post-IR. Body weights were similar in TRPM2+/+ and TRPM2−/− mice and not affected by IR ( Supplementary Fig. S3 ). Further, there was no change in either the morphology of the gland or in the localization of AQP5 and NKCC1 during this period ( Supplementary Figs S4–S6 ). Therefore, we conclude that loss fluid secretion seen in TRPM2+/+ mice is not because of poor health of the animals following IR. Our findings suggest that TRPM2 has a significant contribution to IR-induced irreversible loss of fluid secretion in salivary gland and that loss of TRPM2 induces significant protection of salivary gland function. Possible effects due to neuronal and endothelial cell consequences of IR to salivary gland function cannot be presently excluded [11] . PARP1 mediates activation of TRPM2 by IR It has been well established that PARP1 is activated in cells in response to IR-induced DNA damage leading to the generation of ADPR [20] . Furthermore, PARP1 inhibitors have been shown to block activation of TRPM2 by inhibiting the generation of ADPR, the endogenous ligand for TRPM2 channels [21] . Preincubation of HSG cells with the PARP1 inhibitors, 3-AB (10 μM) or PJ-34 (1 μM) significantly delayed and decreased H 2 O 2 -induced increase in Ca 2+ ( Fig. 5a ). A similar inhibition of IR-induced constitutive Ca 2+ influx was seen in HSG cells treated with these agents ( Fig. 5c ). While the amplitude of [Ca 2+ ] i increase induced by H 2 O 2, as well as IR was decreased by >50% in 3-AB and PJ-34-treated cells compared with untreated control cells, the onset time of [Ca 2+ ] i increase in H 2 O 2 -treated cells increased from 15±4 s in control cells to 165±20 and 149±18 s in 3-AB and PJ-34-treated cells, respectively. Furthermore, peak [Ca 2+ ] i increase was reached in 55±12 s in control cells while it took 150±34 s in 3-AB-treated cells and 225±29 s in cells treated with PJ-34. Consistent with their inhibitory effects on TRPM2-mediated Ca 2+ entry these agents also induced significant increase in the % of viable cells after following 15 Gy-IR of HSG cells ( Supplementary Fig. S7A ). Direct effects of 3-AB and PJ-34 on TRPM2 channel activity can be ruled out based on the lack of effect on ADPR-induced TRPM2 currents ( Supplementary Fig. S7B–E ). In aggregate, these findings suggest that IR-induced activation of TRPM2 is mediated by PARP1. 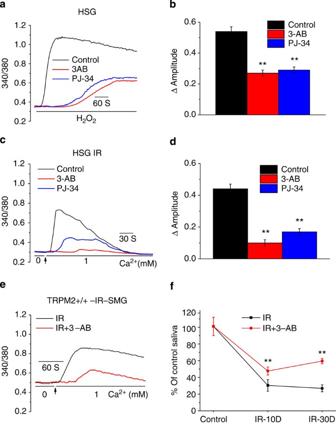Figure 5: PARP inhibitors attenuate IR-induced TRPM2 activation and loss of saliva flow. (a,c) Effect of PARP1 inhibitors 3-AB and PJ-34 (10 and 1 μM, respectively) on H2O2- and IR-induced increases in [Ca2+]iin HSG cells. Cells were incubated with agents for 30 min before H2O2addition or 15 min before IR. Traces are representative data from 225–355 cells. (b,d) Average [Ca2+]ichanges (above basal) calculated from the experiments shown ina,c. **Indicates values that are significantly different (P<0.01, numbers of cells from 265–315) from the respective controls in each case. (e) Constitutive [Ca2+]iincreases in acini isolated from submandibular glands that were excised 24 h after 15 Gy IR. (f) Saliva flow was monitored 10 and 30 day after 15 Gy IR of TRPM2+/+ mice (controls or mice treated with 3-AB, 20 mg kg−1body weight, i.p. injection). Salivary secretion is expressed relative to that measured before IR (**indicates a significant difference (P<0.01) compared with the corresponding values in mice not treated with 3-AB, 10 mice in each group). All values inb,dandfare defined as mean±s.e. Figure 5: PARP inhibitors attenuate IR-induced TRPM2 activation and loss of saliva flow. ( a , c ) Effect of PARP1 inhibitors 3-AB and PJ-34 (10 and 1 μM, respectively) on H 2 O 2 - and IR-induced increases in [Ca 2+ ] i in HSG cells. Cells were incubated with agents for 30 min before H 2 O 2 addition or 15 min before IR. Traces are representative data from 225–355 cells. ( b , d ) Average [Ca 2+ ] i changes (above basal) calculated from the experiments shown in a , c . **Indicates values that are significantly different ( P <0.01, numbers of cells from 265–315) from the respective controls in each case. ( e ) Constitutive [Ca 2+ ] i increases in acini isolated from submandibular glands that were excised 24 h after 15 Gy IR. ( f ) Saliva flow was monitored 10 and 30 day after 15 Gy IR of TRPM2+/+ mice (controls or mice treated with 3-AB, 20 mg kg −1 body weight, i.p. injection). Salivary secretion is expressed relative to that measured before IR (**indicates a significant difference ( P <0.01) compared with the corresponding values in mice not treated with 3-AB, 10 mice in each group). All values in b , d and f are defined as mean±s.e. Full size image Consistent with the results in HSG cells, the constitutive Ca 2+ influx seen in freshly isolated submandibular acinar cells isolated from TRPM2+/+ mice 24 h after 15 Gy IR was significantly reduced in the mice receiving 3-AB (20 mg kg −1 via intraperitoneal (i.p.) injection 1 h before radiation Fig. 5e ). Measurement of salivary gland fluid secretion in 3-AB-treated and untreated TRPM2+/+ mice showed that although both sets of mice displayed an initial loss of salivary fluid secretion those treated with 3-AB retained significantly higher salivary gland function than untreated mice at 10 and 30 days after IR ( Fig. 5f ). A key finding of this study ( Fig. 5f ) was that 3-AB-treated TRPM2+/+ mice displayed significant recovery of fluid secretion, by 30 days after IR there was twofold higher salivary secretion in these mice compared with that in untreated mice. Interestingly, salivary fluid secretion in 3-AB-treated mice at these time points was quite similar to that in IR-TRPM2−/− mice. Thus, 3-AB treatment converted the IR-induced irreversible loss of salivary gland function in TRPM2+/+ mice to a transient, reversible loss, similar to that seen in IR-TRPM2−/− mice. These data provide a link between head and neck IR, production of ADPR via PARP pathway, TRPM2 activation and irreversible loss of salivary gland function. TPL attenuates TRPM2 activation and loss of fluid secretion TPL is a stable nitroxide that has been shown to act a radioprotector in vivo and in vitro [22] , [23] , [24] by several possible mechanisms including oxidizing transition metals, mimicking superoxide dismutase activity and scavenging free radicals. TPL acts on both peroxides and peroxynitrites [22] , [25] , [26] . Pretreatment of HSG cells with 10–100 mM TPL significantly reduced both H 2 O 2 and IR-induced Ca 2+ increases ( Fig. 6a–d ). In addition, pretreatment of HSG cells with 10 mM TPL before 15 Gy IR decreased cell damage ( Supplementary Fig. S2A ). TPL did not exert direct effects on TRPM2 channel activity as shown by lack of change in ADPR-induced TRPM2 currents in TPL-treated cells ( Supplementary Fig. S7C ). Importantly, IR-induced constitutive Ca 2+ influx activity in freshly isolated submandibular acinar cells from TRPM2+/+ mice 24 h after 15 Gy IR was significantly decreased when mice received TPL of 175 mg kg −1 10 min before radiation ( Fig. 6e ). Further, TPL-treated TRPM2+/+ mice showed significant protection of salivary gland function after IR as compared with untreated IR-TRPM2+/+ mice. Although TPL-treated mice also displayed an initial loss of saliva flow, it was 20% greater than that in untreated mice and by 30 days after IR fluid secretion recovered to 70% of initial level, that is, >2-fold higher as compared with the function in untreated mice ( Fig. 6g ). As with 3-AB, TPL also converted the IR-induced irreversible loss of salivary gland function into a relatively transient and reversible loss. 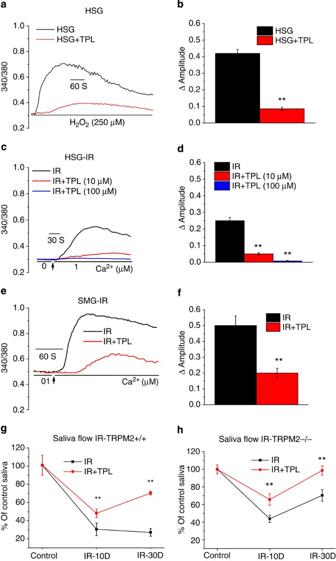Figure 6: TPL attenuates IR-induced TRPM2 activation and decrease in salivary fluid secretion. (a) HSG cells were treated with TPL (10, 100 mM for 10 min) before addition of H2O2. Traces show [Ca2+]ichanges in control and TPL-treated cells. (b) Average values of experiments shown ina. **Indicates a statistically significant difference (P<0.01, number of cells tested from 112–123) compared with unmarked value. (c) Cells were treated with two concentrations of TPL as given ina(10, 100 mM) and then subjected to 15 Gy radiation. [Ca2+]iwas measured within 1 to 1.5 h after IR in IR-HSG and TPL-treated IR cells (average values are given ind). **Indicates values that are significantly different from the control group (P<0.01, number of cells tested from 101–114). (e) Constitutive [Ca2+]iincreases in acini isolated from submandibular glands that were excised 24 h after 15 Gy IR with or without TPL treatment. Average values are given inf(**indicates values that are significantly different from the control group,P<0.01 and number of cells tested from 145–175). (g) Mice were treated with TPL 175 mg kg−1body weight, i.p., 10 min before 15 Gy-IR. SMG were excised and acini were prepared, loaded with fura2 and used for [Ca2+]imeasurements. Traces show representative pattern. (f) Average data from 145–175 cells (from 2–3 mice in each group) are shown. **Indicates values that are significantly different from the control group,P<0.01). TRPM2+/+ mice (g) or TRPM2−/− mice (h) were treated with TPL (175 mg kg−1body weight, i.p., 10 min before 15 Gy-IR) and saliva flow was measured as described above (Fig. 4) on 10 and 30 days after IR. Saliva flow is shown relative to the value obtained before IR (10 animals for TPL-treated group and 29 animals for untreated control, **indicates statistically significant difference,P<0.01 from corresponding values in untreated mice. All values are defined as mean±s.e. inb,dandf–h. Figure 6: TPL attenuates IR-induced TRPM2 activation and decrease in salivary fluid secretion. ( a ) HSG cells were treated with TPL (10, 100 mM for 10 min) before addition of H 2 O 2 . Traces show [Ca 2+ ] i changes in control and TPL-treated cells. ( b ) Average values of experiments shown in a . **Indicates a statistically significant difference ( P <0.01, number of cells tested from 112–123) compared with unmarked value. ( c ) Cells were treated with two concentrations of TPL as given in a (10, 100 mM) and then subjected to 15 Gy radiation. [Ca 2+ ] i was measured within 1 to 1.5 h after IR in IR-HSG and TPL-treated IR cells (average values are given in d ). **Indicates values that are significantly different from the control group ( P <0.01, number of cells tested from 101–114). ( e ) Constitutive [Ca 2+ ] i increases in acini isolated from submandibular glands that were excised 24 h after 15 Gy IR with or without TPL treatment. Average values are given in f (**indicates values that are significantly different from the control group, P <0.01 and number of cells tested from 145–175). ( g ) Mice were treated with TPL 175 mg kg −1 body weight, i.p., 10 min before 15 Gy-IR. SMG were excised and acini were prepared, loaded with fura2 and used for [Ca 2+ ] i measurements. Traces show representative pattern. ( f ) Average data from 145–175 cells (from 2–3 mice in each group) are shown. **Indicates values that are significantly different from the control group, P <0.01). TRPM2+/+ mice ( g ) or TRPM2−/− mice ( h ) were treated with TPL (175 mg kg −1 body weight, i.p., 10 min before 15 Gy-IR) and saliva flow was measured as described above ( Fig. 4 ) on 10 and 30 days after IR. Saliva flow is shown relative to the value obtained before IR (10 animals for TPL-treated group and 29 animals for untreated control, **indicates statistically significant difference, P <0.01 from corresponding values in untreated mice. All values are defined as mean±s.e. in b , d and f – h . Full size image Recovery of fluid secretion in TPL-treated TRPM2−/− mice We examined the combined effect of TPL and lack of TRPM2 activity on IR-induced loss of salivary gland function. TRPM2−/− mice were treated with TPL before radiation and saliva flow was measured at different time point post-IR. Although the pattern of change in salivary fluid secretion was similar in treated and untreated mice, that is, both sets of animals showed initial loss followed by recovery, TPL-treated mice displayed about 30% higher function at both the 10 day and 30 day time points. Remarkably, by 30 days after IR, fluid secretion in TPL-treated TRPM2−/− mice fully recovered to levels similar to that in the mice before IR ( Fig. 6h ). Therefore, it appears that direct, TRPM2-independent, effects of IR account for about 45% of the total irreversible loss of salivary gland function at 120 days after IR, while TRPM2 accounts for about 55% of the loss in saliva flow. (Represents the difference between TRPM2−/− and TRPM2+/+ mice.) This TRPM2-independent loss is almost completely eliminated by TPL treatment of mice before IR. These findings suggest that direct effects of IR, as well as effects mediated via activation of TRPM2 contribute to salivary gland hypofunction. It is important to note that TPL treatment alone does not induce full protection of gland function in TRPM2+/+ mice. One possible explanation for this discrepancy is that TRPM2 somehow amplifies the effects of IR on the gland or contributes to later effects of IR [17] , [19] , [27] , [28] . Effect of 3-AB and TPL on acinar cell volume changes To determine whether effects on acinar cells per se are associated with the reduction in salivary gland fluid secretion, we assessed agonist-stimulated changes in cell volume, which directly reflect acinar cell fluid secretion, by using submandibular gland clusters from TRPM2+/+ mice, control and 60 days after IR ( Fig. 7a ). Cells from control mice displayed a sustained decrease in cell volume following stimulation with 1 μM carbachol (CCh). In contrast, acini from IR-mice showed a transient decrease in cell volume, with >2% decrease in cell volume at 400 s after stimulation (control cells showed ≥30% decrease in volume at this time point). More importantly, cells isolated from mice pretreated with 3-AB or TPL before IR displayed a significant recovery of cell shrinkage with 12.5% and 11.5% volume decrease, respectively; that is, about four to fivefold above that in cells from untreated mice and ~55% less than that in cells from non-irradiated mice ( Fig. 7b ). Together these data demonstrate that effects on acinar cell function per se underlie the recovery of salivary gland fluid secretion in 3-AB- and TPL-treated mice following IR. Furthermore there were not significant differences in agonist-stimulated volume changes of submandibular gland acini (SMG) cells from TRPM−/− mice 2 months after IR compared with matched controls ( Fig. 7c ). 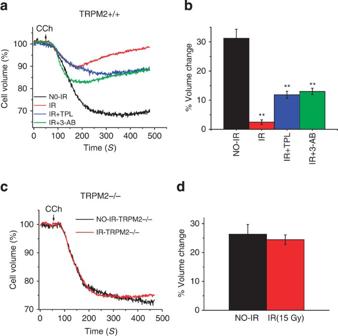Figure 7: 3-AB and TPL mitigate IR-induced loss of acinar cell function. Carbachol (CCh)-induced changes in cell volume were used to assess the secretory function of acinar cells, with decrease in cell volume representing loss of fluid from the cell. SMG cell clusters (see Methods section for details of preparation and assay) were loaded with calcein. Fluorescence was measured with excitation at 488 nm and emission at 510 nm, and expressed relative to initial value (Ft/Fo) in cells prepared from the following groups of TRPM2+/+ mice, control non-irradiated, irradiated (60 days after 15 Gy), mice treated with either 3-AB- or TPL- before IR (as described forFigs 5and6). (a) Traces represent an average of 36–85 regions of interest (ROIs) from four different cell preparations from TRPM2+/+ mice. One micromolar CCh was added where indicated. (b) Average volume change at 400 s after CCh-stimulation, numbers indicate ROI. Data were obtained from four mice for each group. (c) Representative traces from TRPM2−/− mice, control and 2 months after IR. (d) Average volume at 400 s after agonist-activation, numbers of ROI are 38 for IR and 138 for no-IR group and data were obtained from three mice for each group. All values are defined as mean±s.e. inbandd. Figure 7: 3-AB and TPL mitigate IR-induced loss of acinar cell function. Carbachol (CCh)-induced changes in cell volume were used to assess the secretory function of acinar cells, with decrease in cell volume representing loss of fluid from the cell. SMG cell clusters (see Methods section for details of preparation and assay) were loaded with calcein. Fluorescence was measured with excitation at 488 nm and emission at 510 nm, and expressed relative to initial value ( F t / F o ) in cells prepared from the following groups of TRPM2+/+ mice, control non-irradiated, irradiated (60 days after 15 Gy), mice treated with either 3-AB- or TPL- before IR (as described for Figs 5 and 6 ). ( a ) Traces represent an average of 36–85 regions of interest (ROIs) from four different cell preparations from TRPM2+/+ mice. One micromolar CCh was added where indicated. ( b ) Average volume change at 400 s after CCh-stimulation, numbers indicate ROI. Data were obtained from four mice for each group. ( c ) Representative traces from TRPM2−/− mice, control and 2 months after IR. ( d ) Average volume at 400 s after agonist-activation, numbers of ROI are 38 for IR and 138 for no-IR group and data were obtained from three mice for each group. All values are defined as mean±s.e. in b and d . Full size image Cancer therapy regimen that include radiation treatment result in the activation of a number of complex and interrelated signalling events, such as generation of ROS and DNA damage. TRPM2 is the first calcium channel shown to be activated in response to oxidative stress. While other calcium channels, including some TRP channels, are activated by ROS due to direct protein modification, TRPM2 is activated by metabolites generated as a consequence of ROS production in the cell [16] . The activation of TRPM2 by radiation treatment, as well as its possible role in radiation-induced damage to healthy epithelial tissue, has not yet been demonstrated. The major pathways that can be predicted to activate TRPM2 following IR are: (i) ADPR generation due to hydrolysis of NAD + and/or cADPR by glycohydrolases, including the ectoenzymes CD38 and CD157 in the plasma membrane and NADase in the mitochondria [29] , [30] , [31] , [32] or (ii) ADPR generation due to combined action of PARPs (poly(ADPR) polymerases; PARP enzymes) and poly(ADPR) glycohydrolases (PARG enzymes) when hyperactivated in response to DNA damage [33] , [34] , [35] . Herein we report that TRPM2 is activated in salivary gland acinar cells in response to salivary gland IR of mice and significantly contributes to radiation-induced irreversible salivary hypofunction. We show that while control mice display an irreversible loss of salivary gland fluid secretion by 10 days after radiation, TRPM2 knockout mice demonstrate a transient loss of function with significant recovery by 30 days after IR, reaching 70% recovery by 60 days. Consistent with this, acinar cells isolated from irradiated control mice display robust constitutively activated Ca 2+ influx (detected 24 h after IR), which is abrogated in cells from irradiated TRPM2 knockout mice. Together, these findings support our suggestion that TRPM2 activation is an early event after IR and significantly contributes long-term persistent loss of salivary gland function. Although the exact mechanism underlying the loss of salivary gland function following IR has not yet been elucidated, several studies show that there is a slow loss of salivary gland tissue [11] due to likely damage of progenitor cell population within the gland [36] . Notably, although there is no overt loss or disruption of salivary gland tissue at earlier time points, stimulated fluid secretion is severely depressed. While further studies are required to elucidate the molecular basis of these functional changes in the gland, the present findings demonstrate that TRPM2 is activated in salivary gland acinar cells (the site of fluid secretion) as an early response to IR. Importantly, mice that lack TRPM2 recover their salivary function while normal mice undergo an irreversible loss of fluid secretion. Thus, we suggest that TRPM2 is involved in IR-induced irreversible loss of salivary fluid secretion. We cannot exclude the possibility that TRPM2 activation in endothelial or neuronal cells that are present within the gland, and consequent functional damage of those tissues, account for the loss of salivary gland function. While these tissues are present within the salivary glands and have a significant role in the development and function of the gland, their involvement in IR-induced salivary dysfunction has not yet been elucidated. Our data suggest that direct effects of IR (TRPM2-independent), as well as TRPM2-dependent effects contribute to IR-induced loss of salivary gland function. As indicated by our findings the former effects are reversible (as seen in TRPM2−/− mice). We also show that IR-induced TRPM2 activation is mediated by ROS generation, as well as PARP1 activation. 3-AB, a PARP1 inhibitor that blocks activation of TRPM2 by reducing ADPR generation exerted protection of salivary gland function in IR-mice. Further, TPL, a redox-cycling nitroxide that protects several organs, including the heart and brain, from ischaemia/reperfusion damage [37] , [38] , also exerted protection of salivary gland function in IR-mice. The protective effect of TPL was more complete in mice lacking TRPM2. Together, these findings strongly demonstrate that TRPM2 is a potentially important and novel therapeutic target for protection against radiation-induced salivary gland hypofunction. It is important to note that PARP1 inhibitors have generally been used to increase the sensitivity of tumour cells to IR and chemotherapy (primarily via effects on DNA repair mechanisms) [39] , [40] , [41] , [42] , [43] . Furthermore, these agents have been used to protect healthy tissues in conditions where there is ischemia or ROS generation [44] , [45] and as we show here following salivary gland IR. While it is unclear whether PARP inhibitors can differentially affect healthy and tumour cells in the field of IR, TPL selectively protects normal cells from the deleterious effects of IR without affecting the radiation sensitivity of tumour cells [46] . In conclusion, our study provides a strong link between activation of TRPM2 by IR and IR-induced irreversible salivary gland dysfunction. Furthermore, suppression of IR-induced activation of TRPM2 provides significant protection of salivary gland function following IR of mice. Evidence for the involvement of TRPM2 in IR-induced salivary gland dysfunction is provided by the positive effects of TPL and 3-AB, both of which attenuate IR-activation of TRPM2. We propose that antagonists of TRPM2 channel activity, administered alone or in combination with ROS-scavengers, can be potentially important in the protection of salivary gland fluid secretion and prevention of xerostomia in patients receiving radiation treatment for head and neck cancers. Animals and cell culture HSG cells were cultured on glass coverslips with Earle’s minimal essential medium (EMEM). EMEM were supplemented with 10% fetal calf serum, 2 m M glutamine, 1% penicillin/streptomycin at 37 °C in 5% CO 2 . TRPM2+/+ and TRPM2−/− mouse were bred from TRPM2+/− animals (C57BL/6 background) obtained from Kyoto University, Japan and genotyped using the protocol described earlier [47] . TRPM2+/− mice were bred and genotyped using PCR assay. Genomic DNAs were extracted from mouse tail using Wizard’ Genomic DNA purification Kit (Promega, Madison, WI, USA) on day 21. Hundred nonogramof DNA from each mouse was used for PCR reaction with the primers (ROSC1-13F 5′-CTTGGGTTGCAGTCATATGCAGGC-3′, ROSC1-10R 5′-GCCCTCACCATCCGCTTCACGATG-3′ and Pneo5′a 5′-GCCACACGCGTCACCTTAATATGCG-3′. All PCR assays were done in a PerkinElmer Cetus DNA Thermal Cycler (PerkinElmer, Waltham, MA, USA) with conditions as 94 °C for 1 min, 60 °C for 1 min, 72 °C for 1 min for 30 cycles. The 740 bp band was used as the criteria for identification of TRPM2−/− mice. For obtaining samples of salivary glands, mice were euthanized by CO 2 asphyxiation and salivary glands were immediately excised. Breeding and all other procedures were carried out using a protocol approved by the Nation Institute of Dental Craniofacial Research-Animal Care and Use Committee, as well as National Cancer Institute-Animal Care and Use Committee in compliance with the Guide for the Care and Use of Laboratory Animal Resources National Research Council. IR of HSG cells and mice HSG cells at about 70% confluence were irradiated with a dose of 15 Gy using a Pantak X-ray unit at a dose rate of 1.55 Gy min −1 . TRPM2+/+ and TRPM−/− mice (between 8–12 weeks of age, weighing between 16–26 g) were used for IR of salivary glands. Animal were placed into a specially built Lucite jig in such way that the animal could be immobilized without the use of anaesthetics. Additionally, the jig was fitted with a Lucite cone that surrounded the head and prevented head movement during the IR exposure. The jig, with the animals was then covered with a lead shield with apertures to allow IR to target only the areas in the animals where salivary glands are localized. This set-up prevented more general IR of the whole head area [48] . Single IR doses at 15 Gy were delivered by a Therapax DXT300 X-ray irradiator (Pantak Inc., East Haven, CT, USA) using 2-mm Al filtration (300 kVp) at a dose rate of 2.3 Gy min −1 . This IR dose has been established to induce significant (60%) loss of salivary flow in 6–8 weeks after IR [49] . Immediately after IR, animals were removed from the Lucite jig and housed in a climate and light-controlled environment and allowed free access to food and water. All IR animals were fed mouse chow in the form of a gel rather than hard pellets. Salivary Fluid secretion Mice were weighed and anaesthesia was achieved with a solution of ketamine (100 mg ml −1 , Fort Dodge Animal Health, Fort Dodge, IA, USA) and xylazine (20 mg ml −1 , Phoenix, St Joseph, MO, USA) in sterile water by i.p. injection (1 μl g −1 of body weight). Whole saliva was collected after pilocarpine stimulation (0.5 mg kg −1 body weight, administered s.c.). Saliva was collected for up to 20 min after stimulation. Western blot analysis Salivary glands from TRPM2+/+ and −/− mice were excised and homogenized in ice-cold CelLytic M Cell Lysis reagent (Sigma, St Louis, MO, USA). Forty micrograms of protein from each sample was mixed with Tris-Glycine sodium dodecyl sulphate sample buffer (Invitrogen, Grand Island, NY, USA) and loaded onto gels for western blot analysis. Rabbit polyclonal anti-TRPM2 antibody (1:200 dilution, Abcam, Cambridge, MA, USA) and rabbit polyclonal anti-b-actin antibody (1:500 dilution, Abcam) were used for immunoblotting. After incubation with secondary antibodies, signals were detected by chemiluminescence using SuperSignal West Femto Maximum Sensitivity Substrate (Thermo Scientific, Rockford, IL, USA). Localization of TRPM2 in mouse submandibular glands Salivary glands were excised and fixed in 10% formalin and embedded in paraffin. Five micrometre sections of the tissue were blocked with 20% donkey serum (Jackson ImmunoResearch) and then treated with anti-TRPM2 (Abcam) and fluorescein isothiocyanate-labeled secondary antibody. Samples were mounted with vector shield antifade reagent with DAPI (4′,6 diamidino 2 phenylindole; Vector labs) and imaged using a Leica LSM-SP2 confocal microscope. Cell Viability Assay The cell viability was examined using Trypan blue exclusion method. Trypan blue (0.4%) was added to cell suspension and incubated for 5 min at room temperature. Cells were counted using a hemocytometer. The number of viable (unstained) and dead (stained) cells were determined. The number of viable cells is expressed as percentage of total cells (viable+dead). The cell picture was taken using an Olympus microscope with a digital camera using Metamorph software. Whole-cell patch-clamp measurements For patch-clamp experiments, cells were grown on coverslips that were transferred to the recording chamber and bathed in standard extracellular solution composed of (in mM): 145 NaCl, 5 KCl, 10 HEPES, 10 glucose, 1 CaCl 2 , 1 MgCl 2 , pH of 7.4 (adjusted with NaOH) and osmolarity between 305 and 315 mosmol. The patch pipette had resistances between 3–5 MΩ after filling with standard pipette solutions contained (in mM): 140 K-glutamate, 8 NaCl, 1 MgCl 2 , 10 HEPES–KOH. Ca 2+ concentration was buffered to 100 nM. ADPR was added to the pipette solution where indicated. Electrophysiological experiments were performed in the tight-seal whole-cell configuration at room temperature (22–25 °C) using an Axopatch 200B amplifier. Development of the current was monitored by measuring the current amplitudes at a potential of −80 mV, taken from high resolution currents in response to voltage ramps ranging from −90 to 90 mV over a period of 100 ms imposed every 2 s (holding potential was 0 mV) and digitized at a rate of 1 kHz. Liquid-junction potentials were <8 mV and were not corrected. Capacitative currents and series resistance were determined and minimized. For analysis, the current recorded during the first ramp was used for leak subtraction of the subsequent current records. Cell volume measurements in cell cluster preparation Submandibular glands were excised from mice and placed in ice-cold tyrode solution containing (in mM): 130 NaCl, 5.4 KCl, 1CaCl 2, 10 HEPES, 1 MgCl2, 10 glucose, 1% BSA: pH 7.4, that was thoroughly gassed with 95% O 2 5% CO 2 . The glands were finely minced (1 mm pieces) and loaded with 1 μm calcein (Molecular Probes, Invitrogen, Eugene, OR, USA) for 30 min, washed in dye-free tyrode solution for 30 min at room temperature in the dark. Calcein-loaded cell clusters were placed on coverslips, which were coated with Cell Tak (from BD Bioscience, Bedford, MA, USA). The extracellular solution used to place the cluster during experiments included: 130 NaCl, 5.4 KCl, 1CaCl 2, 10 HEPES, 1 MgCl2, 10 glucose, pH 7.4. The coverslip was placed in an open bath chamber and imaged using a Leica SP2 confocal mounted on a DM IRE2 inverted microscope using a × 20 (0.4 NA) dry objective. Images were acquired every 1 s with excitation at 488 nm and emission at 510 nm. Calcein was excited with the 488-nm line of an argon ion laser. Regions of interest were selected, fluorescence intensity was determined as a function of time and expressed relative to the initial fluorescence. As indicated in the figure, cells were stimulated with 1 μm CCh (Sigma, St Louis MO, USA). All experiments were performed at 37 ° C with an incubation chamber mounted to the microscope to maintain temperature. [Ca 2+ ] i Measurements Measurement of [Ca 2+ ] i were performed by imaging Fura-2-loaded cells using an Olympus × 51 microscope (Olympus Centre Valley, PA, USA), with an ORCA-ER camera (Hamamatsu, Tokyo, Japan) attached to a Polychrome V (Till Photonics LLC, Pleasanton, CA, USA). Cells were excited at 340/380 nm and emission was set at 510 nm. Metafluo (Molecular Devices, Downingtown, PA, USA) was used to acquire images and process data. Measurements were made in standard extracellular solution (145 mM NaCl, 5 mM KCl, I mM CaCl 2, 1 mM MgCl 2 , 10 mM HEPES, 10 mM glucose, pH 7.4 (NaOH)). Statistics Data are expressed as mean±s.e. and statistical significance was determined by analysis of variance and * P <0.05 and ** P <0.01 were used to indicate statistically significant. How to cite this article: Liu, X. et al . Loss of TRPM2 function protects against irradiation-induced salivary gland dysfunction. Nat. Commun. 4:1515 doi: 10.1038/ncomms2526 (2013).